Disrupted erythropoietin signalling promotes obesity and alters hypothalamus proopiomelanocortin production Although erythropoietin (Epo) is the cytokine known to regulate erythropoiesis, erythropoietin receptor (EpoR) expression and associated activity beyond haematopoietic tissue remain uncertain. Here we show that mice with EpoR expression restricted to haematopoietic tissues ( Tg ) develop obesity and insulin resistance. Tg -mice exhibit a decrease in energy expenditure and an increase in white fat mass and adipocyte number. Conversely, Epo treatment of wild-type (WT)-mice increases energy expenditure and reduces food intake and fat mass accumulation but shows no effect in body weight of Tg -mice. EpoR is expressed at a high level in white adipose tissue and in the proopiomelanocortin (POMC) neurons of the hypothalamus. Although Epo treatment in WT-mice induces the expression of the polypeptide hormone precursor, POMC, mice lacking EpoR show reduced levels of POMC in the hypothalamus. This study provides the first evidence that mice lacking EpoR in non-haematopoietic tissue become obese and insulin resistant with loss of Epo regulation of energy homeostasis. Obesity occurs when a surplus of body energy is sustained due to an increase in food intake, or decrease in energy expenditure [1] , [2] . Despite growing awareness of obesity worldwide, knowledge of normal physiology of energy homeostasis and fat mass accumulation is still limited. Identifying regulatory factors in energy homeostasis and adipogenesis will provide valuable information for development of effective therapeutic and preventive strategies for human obesity. Erythropoietin (Epo), a cytokine produced in the fetal liver and adult kidney, is required for erythropoiesis [3] . Epo binding to its receptor (EpoR) on erythroid progenitor cells activates Janus kinase 2 and downstream signalling pathways including signal transducer and activator of transcription 5 (STAT5), extracellular-signal-regulated kinase (ERK) and p38 mitogen-activated protein kinase (p38MAPK) [4] , [5] , [6] , [7] , which promote survival, proliferation and differentiation. Mice lacking Epo or EpoR die in utero due to severe anaemia [8] , but also show impaired angiogenesis and defective brain and heart development [9] , [10] , [11] , suggesting Epo activity beyond haematopoietic tissue. A GATA1-promotor/EpoR complementary DNA transgene ( TgEpoR E ) provided erythroid-specific EpoR expression and rescued the phenotype of EpoR −/− mice [12] . These EpoR −/− TgEpoR E ( Tg ) mice had no gross abnormal morphology but showed susceptibility to hypoxia-induced retinopathy of prematurity and to pulmonary hypertension [13] , [14] , suggesting disruption of normal tissue integrity is linked to loss of specific EpoR expression in non-haematopoietic tissue. In this study we found that EpoR expression in wild-type (WT) C57B6 mice was high in white adipose tissue (WAT) and hypothalamus compared with other non-haematopoietic tissues. Tg -mice exhibited significant increase in body weight gain due to increased fat mass and a decrease in total activity and energy expenditure compared with WT-mice. Tg -mice were glucose intolerant and became insulin resistant with the development of obesity. Further analysis demonstrated a regulatory role of Epo in differentiation of preadipocyte cultures and in vivo in adipocyte number, hypothalamus proopiomelanocortin (POMC) expression and energy homeostasis. These observations provide the first evidence for an essential role of endogenous Epo in maintaining normal fat mass in mice. Tg -mice develop obesity Haematopoietic rescue of the EpoR −/− phenotype in Tg -mice overcomes severe anaemia in utero . However, after the first postnatal week we observed a disproportionate increase in body weight. Tg -mice weekly body weight gain was greater by 60% in females and 30% in males compared with WT-mice during the first year, and was due to an increase in fat mass with no change in lean mass ( Fig. 1a–e ). Whole-body X-ray computed tomography (CT) showed a dramatic increase in Tg -mice visceral and subcutaneous white fat ( Fig. 1f–h ). Increased body weight was also observed in a second transgenic line for erythroid rescue of EpoR −/− -mice [12] , indicating that the increase in body weight is not related to transgene insertion site. Although EpoR −/− -mice die in utero , EpoR +/− -mice with or without the transgene ( Fig. 1i,j ) and transgenic mice on a WT background ( EpoR +/+ TgEpoR E ) survive through adulthood with normal haematocrit and no morphological defects [8] , [15] and exhibit normal body weight. 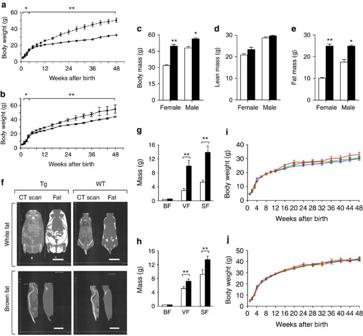Figure 1: EpoR−/−TgEpoREmice (Tg) develop obesity. (a,b) Body weight versus age of WT-mice (solid line) andTg-mice (dashed line) are indicated for female (a) (n=13) and male (b) (n=15) mice. (c–e) Measurements of body weight (c), lean mass (d) and fat mass (e) ofTg-mice (solid bar) and age-/sex-matched WT-mice (open bar) at 8 months of age are indicated (male:Tg(n=4), WT (n=4); female:Tg(n=9), WT (n=6)). (f) Representative whole-body X-ray CT scan of 8-month-old female mice shows fat tissue (white) distribution by density for coronal (upper) views (visceral and subcutaneous white fat) and sagittal (lower) views (brown fat in the dorsal neck), scale bar=20 mm. (g,h) Volume analyses for brown fat (BF), visceral fat (VF) and subcutaneous fat (SF) were determined for female (g) (n=9) and male (h) (n=4) mice. (i,j) Body weight of EpoR heterozygousEpoR+/−-mice (blue) andEpoR+/−TgEpoRE-mice (green) was compared with age-/sex-matched WT-mice (red) (female:iand male:j;n=14 in each group). Error bars indicate s.e.m. and significance is indicated by *P<0.05 and **P<0.01 determined by Student'st-test. Figure 1: EpoR −/− Tg EpoR E mice ( Tg ) develop obesity. ( a,b ) Body weight versus age of WT-mice (solid line) and Tg -mice (dashed line) are indicated for female ( a ) ( n =13) and male ( b ) ( n =15) mice. ( c–e ) Measurements of body weight ( c ), lean mass ( d ) and fat mass ( e ) of Tg -mice (solid bar) and age-/sex-matched WT-mice (open bar) at 8 months of age are indicated (male: Tg ( n =4), WT ( n =4); female: Tg ( n =9), WT ( n =6)). ( f ) Representative whole-body X-ray CT scan of 8-month-old female mice shows fat tissue (white) distribution by density for coronal (upper) views (visceral and subcutaneous white fat) and sagittal (lower) views (brown fat in the dorsal neck), scale bar=20 mm. ( g,h ) Volume analyses for brown fat (BF), visceral fat (VF) and subcutaneous fat (SF) were determined for female ( g ) ( n =9) and male ( h ) ( n =4) mice. ( i,j ) Body weight of EpoR heterozygous EpoR +/− -mice (blue) and EpoR +/− TgEpoR E -mice (green) was compared with age-/sex-matched WT-mice (red) (female: i and male: j ; n =14 in each group). Error bars indicate s.e.m. and significance is indicated by * P <0.05 and ** P <0.01 determined by Student's t -test. Full size image Epo decreases fat mass accumulation Development of obesity in Tg -mice suggested Epo involvement in the regulation of fat mass accumulation. Therefore, we treated adult WT-mice (6 month) fed a high-fat diet (HFD) with high-dose Epo for 3 weeks. Body mass increased <4% in Epo-treated mice with haematocrit increasing up to 80%, but body mass increased more than 18% in saline-treated mice by 3 weeks ( Fig. 2a ). Although lean mass remained the same in both groups, fat mass in saline-treated mice increased by more than 112%, but only by 42% in Epo-treated mice ( Fig. 2b,c ), indicating that Epo treatment greatly suppressed fat mass accumulation. 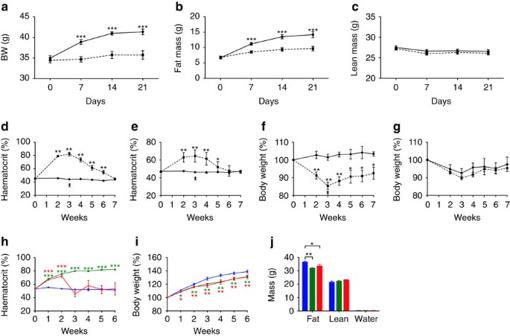Figure 2: Epo treatment decreases fat mass accumulation in WT-mice. (a–c) Male WT-mice (6 months of age) on a HFD were treated with Epo (dashed line) or saline (solid line) (n=8) for 3 weeks. (a) Body weight (BW), fat mass (b) and lean mass (c) were monitored weekly. (d–g) WT- (d,f) andTg-mice (e,g) (8 month of age) fed a normal diet were treated with Epo (dashed line) or saline (solid line) for 3 weeks (n=4). Haematocrit (Hct) (d,e) and body weight (f,g) were monitored weekly for up to 4 weeks after treatment. (h–j) A total of 18 maleob/obmice (12 weeks old) were divided into three groups (n=6 in each group) and placed on HFD for 6 weeks, during which one group was treated with Epo (3000 U kg−1every 2 days) (green) and the other group was treated with the same volume of saline (blue). A third group was treated with Epo and subjected to phlebotomy beginning after 2 weeks to maintain Hct in the normal range (red). Hct (h) and body weight (i) were monitored weekly. Body composition (j) was measured at the end of the 6-week treatment. Error bars indicate s.e.m. and significance is indicated by *P<0.05, **P<0.01 and ***P<0.001 determined by Student'st-test ina–i. Inj, statistical analyses are relative to saline control by one-way analysis of variance (Dunnet's multiple comparison test) and significance is indicated as *P<0.05 and **P<0.01. Figure 2: Epo treatment decreases fat mass accumulation in WT-mice. ( a–c ) Male WT-mice (6 months of age) on a HFD were treated with Epo (dashed line) or saline (solid line) ( n =8) for 3 weeks. ( a ) Body weight (BW), fat mass ( b ) and lean mass ( c ) were monitored weekly. ( d–g ) WT- ( d,f ) and Tg -mice ( e,g ) (8 month of age) fed a normal diet were treated with Epo (dashed line) or saline (solid line) for 3 weeks ( n =4). Haematocrit (Hct) ( d,e ) and body weight ( f,g ) were monitored weekly for up to 4 weeks after treatment. ( h–j ) A total of 18 male ob/ob mice (12 weeks old) were divided into three groups ( n =6 in each group) and placed on HFD for 6 weeks, during which one group was treated with Epo (3000 U kg −1 every 2 days) (green) and the other group was treated with the same volume of saline (blue). A third group was treated with Epo and subjected to phlebotomy beginning after 2 weeks to maintain Hct in the normal range (red). Hct ( h ) and body weight ( i ) were monitored weekly. Body composition ( j ) was measured at the end of the 6-week treatment. Error bars indicate s.e.m. and significance is indicated by * P <0.05, ** P <0.01 and *** P <0.001 determined by Student's t -test in a–i . In j , statistical analyses are relative to saline control by one-way analysis of variance (Dunnet's multiple comparison test) and significance is indicated as * P <0.05 and ** P <0.01. Full size image To determine how haematocrit affects the Epo response in fat mass accumulation, Tg - and WT-mice were treated with Epo for 3 weeks and haematocrit increased from 45% up to ∼ 80% in both WT- and Tg -mice ( Fig. 2d,e ). In WT-mice Epo treatment decreased body weight by 15% compared with a 4% increase with saline treatment ( Fig. 2f ). In contrast, Tg -mice showed no significant difference in body weight between Epo and saline treatment ( Fig. 2g ), suggesting the Epo effect on fat mass accumulation is not related to changes in haematocrit and is dependent on EpoR expression in non-haematopoietic tissues. This was further illustrated when ob/ob -mice were subjected to phlebotomy beginning after 2 weeks of Epo treatment to maintain the haematocrit in the normal range ( Fig. 2h ). Body weight gain and fat mass accumulation in ob/ob -mice treated with Epo were similar with and without phlebotomy and were significantly decreased compared with saline treatment ( Fig. 2i,j ). With increased fat mass, Tg -mice also showed increased plasma insulin levels ( Fig. 3a,b ). Glucose intolerance was identified by 2 months ( Fig. 3c–e ). At 8 months fasting plasma insulin levels, plasma triglyceride and fasting blood glucose were significantly greater than those in WT-mice ( Fig. 3f–h ). Tg -mice also showed exacerbated glucose intolerance and a markedly blunted response to insulin stimulation despite a significantly elevated insulin level ( Fig. 3i,j ). The increase in body fat and resultant obesity preceded the onset of insulin resistance ( Supplementary Fig. S1 ), suggesting a type 2 diabetes-like phenotype. In comparison, EpoR +/− - and EpoR +/− TgEpoR E -mice did not become obese ( Fig. 1i,j ) and exhibited normal glucose and insulin tolerance at 6 and 12 months. Interestingly, in WT-mice (3 months) fed HFD, Epo treatment for 6 weeks reduced fat mass accumulation, fasting plasma glucose and insulin levels, and glucose stimulated insulin secretion, and improved glucose tolerance ( Supplementary Fig. S2 ). 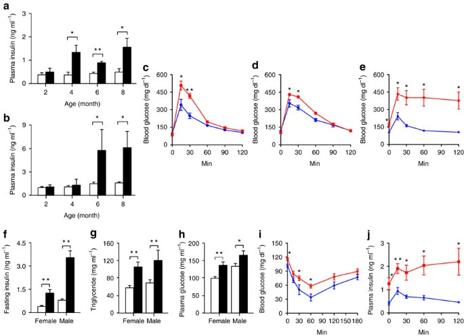Figure 3: Metabolic changes inTg-mice. (a,b) Plasma insulin levels were measured inTg(solid bar) and WT (open bar) age-matched female (a) and male (b) mice (n=9). (c,d) Glucose tolerance test (GTT) was performed inTg-mice (red line) and age-matched WT-mice (blue line) at 2 months (female:c; male:d,n=5 in each group). (e) GTT on femaleTg-mice (red line) (n=9) and WT-mice (blue line) (n=5) at age of 8 month. (f–h) Fasting plasma insulin (f), plasma triglyceride (g) and fasting blood glucose (h) were determined forTg-mice (solid bar) and WT-mice (open bar) at age of 8 months (female:Tg(n=10), WT (n=4); male:Tg(n=5), WT (n=4)). (i) Insulin tolerance test on femaleTg-mice (red line) (n=9) and WT-mice (blue line) (n=5) at age of 8 month. (j) Plasma insulin concentration after glucose stimulation was determined using radioimmunoassay for femaleTg- (red line) and WT-mice (blue line) at 8 months of age (Tg(n=9); WT (n=5)). Error bars indicate s.e.m. and significance is indicated by *P<0.05 and **P<0.01 determined by Student'st-test. Figure 3: Metabolic changes in Tg -mice. ( a,b ) Plasma insulin levels were measured in Tg (solid bar) and WT (open bar) age-matched female ( a ) and male ( b ) mice ( n =9). ( c,d ) Glucose tolerance test (GTT) was performed in Tg -mice (red line) and age-matched WT-mice (blue line) at 2 months (female: c ; male: d , n =5 in each group). ( e ) GTT on female Tg -mice (red line) ( n =9) and WT-mice (blue line) ( n =5) at age of 8 month. ( f–h ) Fasting plasma insulin ( f ), plasma triglyceride ( g ) and fasting blood glucose ( h ) were determined for Tg -mice (solid bar) and WT-mice (open bar) at age of 8 months (female: Tg ( n =10), WT ( n =4); male: Tg ( n =5), WT ( n =4)). ( i ) Insulin tolerance test on female Tg -mice (red line) ( n =9) and WT-mice (blue line) ( n =5) at age of 8 month. ( j ) Plasma insulin concentration after glucose stimulation was determined using radioimmunoassay for female Tg - (red line) and WT-mice (blue line) at 8 months of age ( Tg ( n =9); WT ( n =5)). Error bars indicate s.e.m. and significance is indicated by * P <0.05 and ** P <0.01 determined by Student's t -test. Full size image Epo regulation of energy homeostasis Although no differences in body temperature or food intake were observed when Tg - and WT-mice were on a regular diet, body weight gain normalized to food intake was significantly higher in Tg -mice ( Supplementary Fig. S3a–c ), suggesting decreased energy expenditure in Tg -mice. We assessed locomotor activity and metabolic rate in young Tg -mice (2–3 months) before development of noticeable obesity. Tg -mice were less active, showed significantly decreased total moving distance and total movement time, and increased total resting time in the open-field test ( Fig. 4a–c ). An indirect calorimetry study showed decreased total activity in Tg -mice and reduced total oxygen consumption and respiratory quotient ( Fig. 4d,e ; Supplementary Fig. S3d,e ). Energy efficiency in Tg -mice was significantly higher than that of WT-mice ( Fig. 4f ). Similarly, when mice were fed a HFD, although cumulative food intake was comparable between WT- and Tg -mice, locomotor activity, oxygen consumption and respiratory quotient in Tg -mice were significantly lower and energy efficiency was markedly higher ( Fig. 4g–j ; Supplementary Fig. S3f,g ). 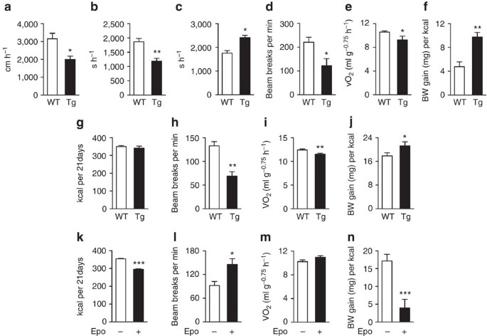Figure 4: Locomotor activity and energy expenditure inTg-mice and Epo-treated WT-mice. (a–f)Tg-mice (n=5, female) and WT-mice (n=9, female) at age of 2 month were compared. Total moving distance (a), total moving time (b) and total rest time (c) in open-field assay and total activity (d) and total oxygen consumption (normalized to the allometrically corrected body weight) (e) in indirect calorimetry assay are presented. Energy efficiency (f) indicates body weight gain versus accumulative energy intake during a 3-week time period. (g–j) Indirect calorimetry assay was performed on 6-month-old WT-mice andTg-mice (n=8, female) during 3 weeks of HFD. Cumulative energy intake (g), total activity (h), normalized total oxygen consumption (i) and energy efficiency (j) were compared. (k–n) In a separate experiment, male WT-mice at age of 6 month were treated with Epo or saline (n=8) during 3 weeks of HFD. Cumulative food intake (k), total activity (l), normalized total oxygen consumption (m) and energy efficiency (n) were determined by indirect calorimetry assay during this period. Error bars indicate s.e.m. and significance is indicated as *P<0.05, **P<0.01 and ***P<0.001 determined by Student'st-test. Figure 4: Locomotor activity and energy expenditure in Tg -mice and Epo-treated WT-mice. ( a–f ) Tg -mice ( n =5, female) and WT-mice ( n =9, female) at age of 2 month were compared. Total moving distance ( a ), total moving time ( b ) and total rest time ( c ) in open-field assay and total activity ( d ) and total oxygen consumption (normalized to the allometrically corrected body weight) ( e ) in indirect calorimetry assay are presented. Energy efficiency ( f ) indicates body weight gain versus accumulative energy intake during a 3-week time period. ( g–j ) Indirect calorimetry assay was performed on 6-month-old WT-mice and Tg -mice ( n =8, female) during 3 weeks of HFD. Cumulative energy intake ( g ), total activity ( h ), normalized total oxygen consumption ( i ) and energy efficiency ( j ) were compared. ( k–n ) In a separate experiment, male WT-mice at age of 6 month were treated with Epo or saline ( n =8) during 3 weeks of HFD. Cumulative food intake ( k ), total activity ( l ), normalized total oxygen consumption ( m ) and energy efficiency ( n ) were determined by indirect calorimetry assay during this period. Error bars indicate s.e.m. and significance is indicated as * P <0.05, ** P <0.01 and *** P <0.001 determined by Student's t -test. Full size image In comparison, Epo treatment of WT-mice on HFD significantly reduced food intake of each WT-mouse ( Fig. 4k ), suggesting that the Epo effect on regulating food intake is dose dependent. These mice exhibited significantly increased locomotor activity ( Fig. 4l ) and resting oxygen consumption (by 9.2%, P =0.01, Student's t -test) whereas their rectal temperature was unchanged. Total oxygen consumption showed an increasing trend compared with saline-treated counterparts ( Fig. 4m ; Supplementary Fig. S3h,i ). Epo treatment also decreased energy efficiency by fourfold ( Fig. 4n ), whereas energy efficiency increased in Tg -mice with restricted Epo response. In both Tg -mice and Epo-treated WT-mice, disrupted Epo signalling equilibrium led to a breakdown in energy homeostasis. Although an Epo-induced increase in muscular fat oxidation by supra-physiologic levels of Epo has been suggested [16] , its effect in regulating energy homeostasis may be critical in the development of obesity in Tg -mice and in suppressed fat mass accumulation in Epo-treated WT-mice. Epo and expression of leptin and adiponectin Leptin and adiponectin, adipokines secreted by WAT, regulate endogenous glucose production, fatty acid oxidation and food intake through binding to their specific receptors in target organs such as the brain, liver and muscle [17] , [18] . Serum leptin levels were higher in Tg -mice and reduced in Epo-treated WT-mice compared with control WT-mice, and seemed proportional to WAT mass whereas leptin mRNA levels were unchanged in WAT of these animals ( Fig. 5a–e ). Similarly, Tg -mice at a younger age (before 4 month) showed significantly higher serum adiponectin levels and no changes in their mRNA levels compared with WT-mice ( Fig. 5e,f ). In contrast, Epo-treated WT-mice showed markedly lower serum adiponectin level compared with control WT-mice ( Fig. 5g ). Furthermore, Epo treatment (24 h) did not change leptin and adiponectin gene expression in both undifferentiated (d0) and differentiated (d7) WT-mouse embryonic fibroblast (MEF) cells ( Fig. 5h,i ). These results suggest that Epo has no effect on leptin and adiponectin gene expression. As Epo treatment of ob/ob -mice significantly decreased fat mass accumulation compared with saline-treated counterparts ( Fig. 5j ), the Epo effect on fat mass accumulation was not dependent on leptin activity. 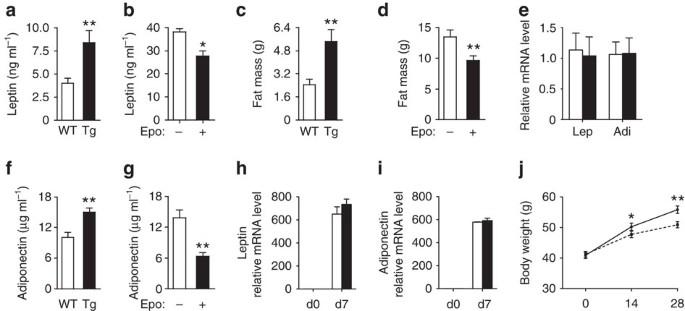Figure 5: Leptin and adiponectin inTg-mice and Epo-treated WT-mice. (a,c,e,f) Serum leptin level (a), fat mass (c), leptin and adiponectin mRNA level in WAT (e) and serum adiponectin level in (f)Tg-mice (solid bar) and WT-mice (open bar) (female,n=8) were compared at age of 4 month. (b,d,g) The 6 month-old WT-mice on HFD were treated with Epo (solid bar) or saline (open bar) (male,n=8) for 3 weeks; serum leptin level (b), fat mass (d) and serum adiponectin level (g) were determined at the end of treatment. (h,i) WT-MEF cells before (d0) and after differentiation (d7) were treated with (closed bar) and without (open bar) Epo (5 U ml−1). Leptin (h) and adiponectin (i) expression was analysed using quantitative real time PCR after 24 h. (j) The 4-month-oldob/ob-mice (male) on HFD were treated with Epo (dashed line) or saline (solid line) for 4 weeks (n=6) and body weights were monitored. Error bars indicate s.e.m. and significance is indicated as *P<0.05 and **P<0.01 determined by Student'st-test. Figure 5: Leptin and adiponectin in Tg -mice and Epo-treated WT-mice. ( a,c,e,f ) Serum leptin level ( a ), fat mass ( c ), leptin and adiponectin mRNA level in WAT ( e ) and serum adiponectin level in ( f ) Tg -mice (solid bar) and WT-mice (open bar) (female, n =8) were compared at age of 4 month. ( b,d,g ) The 6 month-old WT-mice on HFD were treated with Epo (solid bar) or saline (open bar) (male, n =8) for 3 weeks; serum leptin level ( b ), fat mass ( d ) and serum adiponectin level ( g ) were determined at the end of treatment. ( h,i ) WT-MEF cells before (d0) and after differentiation (d7) were treated with (closed bar) and without (open bar) Epo (5 U ml −1 ). Leptin ( h ) and adiponectin ( i ) expression was analysed using quantitative real time PCR after 24 h. ( j ) The 4-month-old ob/ob -mice (male) on HFD were treated with Epo (dashed line) or saline (solid line) for 4 weeks ( n =6) and body weights were monitored. Error bars indicate s.e.m. and significance is indicated as * P <0.05 and ** P <0.01 determined by Student's t -test. Full size image We examined the expression of other adipokines in WAT of WT-, Tg - and ob/ob -mice and observed increased expression of proinflammatory adipokines, Ccl1 and tumour-necrosis factor-α, decreased expression of NOS2 (iNOS) and no change in Csf1 (M-CSF), IL-1β and IL-6 expression in both Tg - and ob/ob -mice compared with WT control mice ( Supplementary Fig. S4 ). Interestingly, we found reduced IL-10 expression in Tg -WAT. The increase in proinflammatory adipokines and decrease in IL-10 raises the possibility that loss of EpoR in non-haematopoietic tissue contributes to increased inflammation giving rise to insulin resistance. Epo effect on preadipocyte differentiation EpoR gene expression was analysed in multiple tissues including white fat, brown fat, liver, kidney, muscle, heart and spleen ( Fig. 6a ). Spleen, a haematopoietic tissue in mice, exhibited the highest level of EpoR expression. Unexpectedly, a high level of EpoR expression (60% of spleen) was observed in WAT. In comparison, EpoR expression in other non-haematopoietic tissues was no greater than 10% the level in spleen. Analysis of WAT fractions from inguinal fat pads of WT-mice showed comparable EpoR expression between stromal vascular cells and adipocytes ( Fig. 6b ). 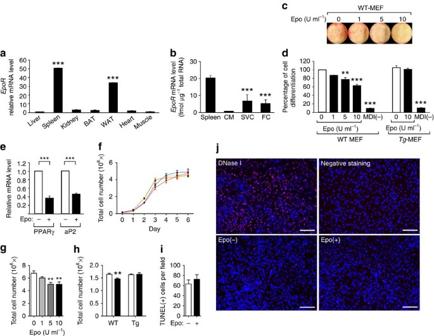Figure 6: EpoR expression and Epo inhibition of preadipocyte differentiation. (a) EpoR mRNA levels in tissues from WT-mice (male,n=3) as indicated including brown adipose tissue (BAT) and WAT were quantified using SYBR green real-time RT–PCR and presented as fold changes relative to mRNA level in liver. (b) Absolute amount of EpoR mRNA in spleen, neonatal cardiomyocytes (CM) and WAT stromal vascular cells (SVC) and fat cells (FC) (n=3) was determined using Taqman PCR. (c) WT-MEF cells treated with Epo at concentrations as indicated were stained with oil red O at the end of differentiation (day 9). (d) Quantification of oil red O staining in differentiated WT-MEF andTg-MEF cultures was presented as percentage relative to WT-MEF culture without Epo. MDI(−) indicates cultures without differentiation induction. (e) Relative PPARγ and aP2 mRNA levels in 3T3-L1 cells without and with Epo treatment (5 U ml−1) during differentiation (day 6). (f) 3T3-L1 cells (1.5×105/well) were cultured with Epo at 0 (circle, blue-line), 1 (square, green-line), 5 (triangle, yellow-line) and 10 U ml−1(inverted-triangle, red-line) until reaching full confluence at day 6. Cells were counted daily using Countess automated cell counter (Invitrogen) in three replicate experiments. (g) 3T3-L1 cells were cultured for 2 days after reaching confluence and then for 3 days in differentiation induction medium (MDI) with Epo at concentrations as indicated. Cells were counted at day 3 (three replicate experiments). (h) Similarly, WT- andTg-MEF cells were cultured in MDI with or without Epo (5 U ml−1), and cells were counted at day 3 (three replicate experiments). (i–j) 3T3-L1 cells were cultured as described ingand assessed with TUNEL staining at day 3. TUNEL(+) cells were counted in 20 randomly selected fields (×200) from each well (six-well plate) of three wells in total for each condition (i). The positive control were treated with DNase I before application of TUNEL staining, and the negative control was stained without terminal deoxynucleotidyl transferase (j). Scale bar=100 μm. Error bars indicate s.e.m. and significance is indicated as **P<0.01 and ***P<0.001 determined by one-way analysis of variance (Dunnet's multiple comparison test) (a,b,d,g) and Student'st-test (e,h). Figure 6: EpoR expression and Epo inhibition of preadipocyte differentiation. ( a ) EpoR mRNA levels in tissues from WT-mice (male, n =3) as indicated including brown adipose tissue (BAT) and WAT were quantified using SYBR green real-time RT–PCR and presented as fold changes relative to mRNA level in liver. ( b ) Absolute amount of EpoR mRNA in spleen, neonatal cardiomyocytes (CM) and WAT stromal vascular cells (SVC) and fat cells (FC) ( n =3) was determined using Taqman PCR. ( c ) WT-MEF cells treated with Epo at concentrations as indicated were stained with oil red O at the end of differentiation (day 9). ( d ) Quantification of oil red O staining in differentiated WT-MEF and Tg -MEF cultures was presented as percentage relative to WT-MEF culture without Epo. MDI(−) indicates cultures without differentiation induction. ( e ) Relative PPARγ and aP2 mRNA levels in 3T3-L1 cells without and with Epo treatment (5 U ml −1 ) during differentiation (day 6). ( f ) 3T3-L1 cells (1.5×10 5 /well) were cultured with Epo at 0 (circle, blue-line), 1 (square, green-line), 5 (triangle, yellow-line) and 10 U ml −1 (inverted-triangle, red-line) until reaching full confluence at day 6. Cells were counted daily using Countess automated cell counter (Invitrogen) in three replicate experiments. ( g ) 3T3-L1 cells were cultured for 2 days after reaching confluence and then for 3 days in differentiation induction medium (MDI) with Epo at concentrations as indicated. Cells were counted at day 3 (three replicate experiments). ( h ) Similarly, WT- and Tg -MEF cells were cultured in MDI with or without Epo (5 U ml −1 ), and cells were counted at day 3 (three replicate experiments). ( i–j ) 3T3-L1 cells were cultured as described in g and assessed with TUNEL staining at day 3. TUNEL(+) cells were counted in 20 randomly selected fields (×200) from each well (six-well plate) of three wells in total for each condition ( i ). The positive control were treated with DNase I before application of TUNEL staining, and the negative control was stained without terminal deoxynucleotidyl transferase ( j ). Scale bar=100 μm. Error bars indicate s.e.m. and significance is indicated as ** P <0.01 and *** P <0.001 determined by one-way analysis of variance (Dunnet's multiple comparison test) ( a,b,d,g ) and Student's t -test ( e,h ). Full size image High EpoR expression in WAT of WT-mice (WT-WAT) and increased white fat mass in Tg -mice ( Tg -WAT) that lack EpoR expression in WAT led us to hypothesize that Epo signalling may affect adipogenesis. Primary MEF cells were induced to differentiate into adipocytes by treatment with 3-isobutyl-1-methylxanthine, dexamethasone and insulin (MDI) for 3 days followed by insulin supplementation. Epo addition to MEF cultures from WT-mice (WT-MEF) decreased preadipocyte differentiation by 23% at 5 U ml −1 and by 37% at 10 U ml −1 , determined by oil red O staining ( Fig. 6c,d ). In comparison, differentiation of MEF cells from Tg -mice ( Tg -MEF) was unaffected by Epo treatment and comparable to WT-MEF cells without Epo ( Fig. 6d ). In 3T3-L1 cells, Epo treatment reduced preadipocyte differentiation and PPARγ and aP2 expression ( Fig. 6e ). Further analysis showed although Epo did not affect 3T3-L1 proliferation in standard culture media, Epo reduced the terminal expansion of cell number (by 25%) obtained with induction of adipocyte differentiation by MDI ( Fig. 6f,g ). Epo also decreased the terminal expansion of WT-MEF cell number (by 14%) during induction of preadipocyte differentiation but not in Tg -MEF cultures ( Fig. 6h ). Both TUNEL and flow cytometry analysis showed this Epo effect was not due to increased cell death ( Fig. 6i,j ; Supplementary Fig. S5 ). These results demonstrate that Epo has a significant effect in reducing preadipocyte expansion during differentiation induction in culture. To assess the mechanism of Epo activity, we examined the potential EpoR downstream signalling molecules, such as STAT5a, ERK and p38MAPK. Activation of MAPKs has been shown to inhibit the activity of PPARγ, a master regulator of adipogenesis [19] . Both expression and phosphorylation of ERK44/42, p38MAPK and PPARγ were comparable in WT-MEF and Tg -MEF cells under normal culture conditions ( Supplementary Fig. S6a ). Epo treatment of WT-MEF cells during differentiation, but not in Tg -MEF cells, induced significant increase in phosphorylation of ERK42 (p-ERK42), ERK 44 (p-ERK44) and p38MAPK (P-p38MAPK) and led to an increase in PPARγ phosphorylation (p-PPARγ) at day 7 and 9, whereas overall expression levels remained comparable ( Fig. 7a ; Supplementary Fig. S6b ). STAT5a expression increased significantly during late adipocyte differentiation, as previously reported [20] , but showed no difference between WT- and Tg -MEF cells ( Supplementary Fig. S6c,d ). PPARγ phosphorylation induced by Epo stimulation suggests that Epo may regulate PPARγ phosphorylation through ERK and p38MAPK signalling pathways during preadipocyte differentiation. 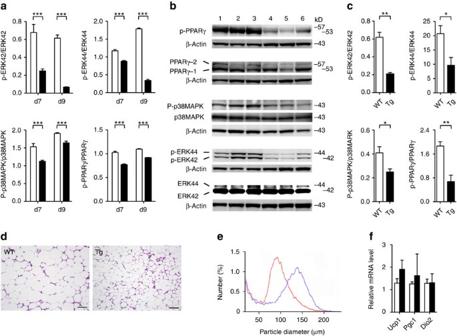Figure 7: Epo effects in preadipocytes during differentiation and WAT fromTg-mice. (a) Western blotting was performed on MEF cells from WT-mice (open bar) andTg-mice (closed bar) cultured with Epo under differentiation inducing condition for 9 days. Results were quantitatively assessed for the expression and phosphorylation (p-) of ERK42, ERK44, p38MAPK and PPARγ, and presented as the ratio of phosphorylation to total expression at day 7 (d7) and 9 (d9). Data were obtained from three replicate experiments. (b,c) Western blotting (b) and quantitative analysis (c) for the expression and phosphorylation (p-) of ERK42, ERK44, p38MAPK and PPARγ were performed on WAT from WT- (open bar) (n=3) andTg-mice (closed bar) (n=3). Results were presented as the ratio of phosphorylation to total expression. Each lane in the western blot represents WAT collected from a different mouse. (d) Representative haematoxylin and eosin staining of gonadal fat pad sections from WT-mice (WT) andTg-mice (Tg) at age of 8 month. Scale bar=100 μM. (e) Direct analysis of adipocyte cell size in WAT by Beckman Coulter Multisizer indicates that the cell size inTg-mice (50%: 95.9 μm diameter) (red) is smaller than in WT mice (50%: 129.5 μm diameter) (blue). (f) Expression of mUcp1, mpgc1 and mDio2 in brown adipose tissue from WT-mice (open bar) andTg-mice (closed bar) (female,n=8) at age of 6 months was determined using quantitative real time RT-PCR with normalization to 18S. Error bars indicate s.e.m. and significance is indicated as *P<0.05, **P<0.01 and ***P<0.001 determined by Student'st-test. Figure 7: Epo effects in preadipocytes during differentiation and WAT from Tg -mice. ( a ) Western blotting was performed on MEF cells from WT-mice (open bar) and Tg -mice (closed bar) cultured with Epo under differentiation inducing condition for 9 days. Results were quantitatively assessed for the expression and phosphorylation (p-) of ERK42, ERK44, p38MAPK and PPARγ, and presented as the ratio of phosphorylation to total expression at day 7 (d7) and 9 (d9). Data were obtained from three replicate experiments. ( b,c ) Western blotting ( b ) and quantitative analysis ( c ) for the expression and phosphorylation (p-) of ERK42, ERK44, p38MAPK and PPARγ were performed on WAT from WT- (open bar) ( n =3) and Tg -mice (closed bar) ( n =3). Results were presented as the ratio of phosphorylation to total expression. Each lane in the western blot represents WAT collected from a different mouse. ( d ) Representative haematoxylin and eosin staining of gonadal fat pad sections from WT-mice (WT) and Tg -mice (Tg) at age of 8 month. Scale bar=100 μM. ( e ) Direct analysis of adipocyte cell size in WAT by Beckman Coulter Multisizer indicates that the cell size in Tg -mice (50%: 95.9 μm diameter) (red) is smaller than in WT mice (50%: 129.5 μm diameter) (blue). ( f ) Expression of mUcp1, mpgc1 and mDio2 in brown adipose tissue from WT-mice (open bar) and Tg -mice (closed bar) (female, n =8) at age of 6 months was determined using quantitative real time RT-PCR with normalization to 18S. Error bars indicate s.e.m. and significance is indicated as * P <0.05, ** P <0.01 and *** P <0.001 determined by Student's t -test. Full size image Epo effect on WAT Since Epo stimulation activates ERK and p38MAPK signalling pathways in differentiating preadipocytes, we speculate that ablation of EpoR would reduce the activity of these signalling pathways in WAT. Indeed, differences in WAT from WT- and Tg -mice were analogous to those observed in MEF cells. Phosphorylation of p38MAPK, ERK44, ERK42 and PPARγ in Tg -WAT was significantly lower than in WT-WAT, although protein expression levels were unchanged ( Fig. 7b,c ). These results suggest a role of Epo in regulating MAPKs activity and PPARγ phosphorylation in WAT. Assessment of adipocyte size distribution in gonadal fat pads showed a shift to smaller cells despite a marked increase in white fat mass in Tg -mice. Consistent with the histological characteristics revealed in tissue sections, direct analysis of adipocyte size in WAT by flow cytometry provided further evidence that fat cell size in Tg -mice is smaller than in WT-mice ( Fig. 7d,e ). The increase in adipocyte number in Tg -WAT compared with WT-WAT is consistent with preadipocyte culture studies where preadipocyte differentiation and cell number increased in the absence of Epo stimulation. In contrast to high EpoR expression in WAT, we detected only a low level of EpoR in brown fat and no differences in PPARγ expression and phosphorylation or in Epo signalling in brown adipose tissues from WT- and Tg -mice. Similarly, no alterations in mRNA levels of BAT-specific genes, Ucp1 , Pgc1α and Dio2 , were found between WT- and Tg -mice ( Fig. 7f ), suggesting that BAT is not Epo responsive. Epo stimulation of POMC expression Decreased locomotor activity and energy expenditure in Tg -mice, and decreased food intake and increased locomotor activity and energy expenditure in WT-mice with Epo treatment suggested that Epo contributes to the central regulation of energy homeostasis. We found high a level of EpoR expression in hypothalamus comparable to WT-WAT ( Fig. 8a ). EpoR expression was increased in WAT from WT-mice on HFD and ob/ob -mice ( Supplementary Fig. S7 ), but absent in Tg -WAT, indicating that EpoR expression in WAT does not generally correlate directly with fat mass accumulation, which is primarily related to changes in energy homeostasis. However, EpoR expression in the hypothalamus was absent in Tg -mice and significantly reduced in ob/ob -mice compared with littermate control and WT-mice ( Fig. 8b ), suggesting an inverse relationship with fat mass accumulation. Gene expression analysis of hypothalamic neuropeptides, that regulates activity, food intake and energy homeostasis [21] , revealed that expression of POMC decreased more than 50% in Tg -mice compared with WT-mice whereas comparable levels of expression were observed for agouti-related protein (AGRP), neuropeptide Y (NPY), melanin-concentrating hormone (pro-MCH) and prepro-orexin ( Fig. 8c ). Furthermore, Epo treatment in WT-mice increased POMC mRNA by threefold, but had no effect on hypothalamic expression of NPY, AGRP, pro-MCH and prepro-orexin ( Fig. 8d ). Immunostaining for EpoR on WT-mouse brain sections revealed specific staining on neurons in the hypothalamus that were identified to be exclusively POMC neurons by double immunostaining ( Fig. 8e ). These findings led us to speculate that in the brain, Epo directly stimulates POMC neurons to induce α-melanocyte-stimulating hormone production that acts through binding to melanocortin receptor MC3R and MC4R, and exerts a direct effect on food intake and energy homeostasis [22] . To confirm that Epo can directly regulate POMC gene expression, adult hypothalamic neurons were prepared and cultured with or without Epo for 24 h. Epo treatment increased POMC gene expression by fourfold, but did not change the gene expression level of NPY, AGRP, pro-MCH and prepro-orexin ( Fig. 8f ). These data suggest that EpoR expression in POMC neurons permits a direct response to exogenous Epo stimulation. Thus, affecting energy homeostasis by increasing POMC production in the hypothalamus of WT-mice and obese mice, albeit at a lower level, but not in Tg -mice that lack EpoR in the hypothalamus. 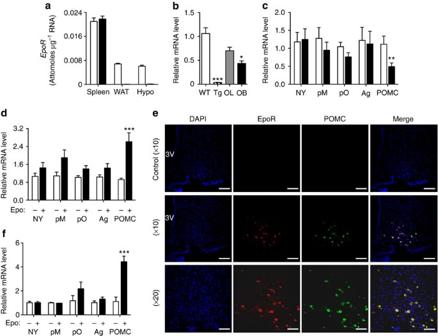Figure 8: Epo regulation of hypothalamic neuropeptide expression. (a) Absolute quantification of EpoR mRNA in spleen, WAT and hypothalamus (Hypo) from WT- (open bar) andTg-mice (closed bar) at age of 6 months (female,n=8) was determined by Taqman PCR. (b) Relative EpoR expression in Hypo from WT- andTg-mice (male,n=5) at age of 6 months, andob/ob-mice (OB) and lean littermates (OL) (male,n=6) at age of 4 months was determined by SYBR green RT-PCR. (c) Expression of NPY (NY), Pro-MCH (pM), prepro-orexin (pO), AGRP (Ag) and POMC in Hypo from WT-mice (open bar) andTg-mice (closed bar) (female,n=8) at age of 6 months was determined by SYBR green RT–PCR. (d) Expression of NY, pM, pO, Ag and POMC in Hypo from 6-month-old WT-mice treated with Epo (closed bar) or saline (open bar) (male,n=8) for 3 weeks was similarly determined. (e) Double fluorescent immunostaining for EpoR (red) and POMC (green) on coronal Hypo sections was combined with DAPI staining (blue) for nuclei. The top panel shows the staining without adding primary antibodies as negative control. Scale bar in the top and middle panels: 100 μm. Scale bar in the bottom panel: 50 μm (3 V indicates third ventricle). (f) Adult neurons isolated from WT Hypo were cultured for 24 h and then stimulated with Epo (5 U ml−1) or saline for 24 h. Total RNA was isolated after Epo or saline treatment and analysed for NY, pM, pO, Ag and POMC expression using quantitative real time PCR. Error bars indicate s.e.m. and significance is indicated as *P<0.05, **P<0.01 and ***P<0.001 determined by Student'st-test inc,dandf. Statistical analyses inbare relative to WT-WAT by one-way analysis of variance (Dunnet's multiple comparison test) and significance is indicated as *P<0.05 and ***P<0.001. Figure 8: Epo regulation of hypothalamic neuropeptide expression. ( a ) Absolute quantification of EpoR mRNA in spleen, WAT and hypothalamus (Hypo) from WT- (open bar) and Tg -mice (closed bar) at age of 6 months (female, n =8) was determined by Taqman PCR. ( b ) Relative EpoR expression in Hypo from WT- and Tg -mice (male, n =5) at age of 6 months, and ob/ob -mice (OB) and lean littermates (OL) (male, n =6) at age of 4 months was determined by SYBR green RT-PCR. ( c ) Expression of NPY (NY), Pro-MCH (pM), prepro-orexin (pO), AGRP (Ag) and POMC in Hypo from WT-mice (open bar) and Tg -mice (closed bar) (female, n =8) at age of 6 months was determined by SYBR green RT–PCR. ( d ) Expression of NY, pM, pO, Ag and POMC in Hypo from 6-month-old WT-mice treated with Epo (closed bar) or saline (open bar) (male, n =8) for 3 weeks was similarly determined. ( e ) Double fluorescent immunostaining for EpoR (red) and POMC (green) on coronal Hypo sections was combined with DAPI staining (blue) for nuclei. The top panel shows the staining without adding primary antibodies as negative control. Scale bar in the top and middle panels: 100 μm. Scale bar in the bottom panel: 50 μm (3 V indicates third ventricle). ( f ) Adult neurons isolated from WT Hypo were cultured for 24 h and then stimulated with Epo (5 U ml −1 ) or saline for 24 h. Total RNA was isolated after Epo or saline treatment and analysed for NY, pM, pO, Ag and POMC expression using quantitative real time PCR. Error bars indicate s.e.m. and significance is indicated as * P <0.05, ** P <0.01 and *** P <0.001 determined by Student's t -test in c , d and f . Statistical analyses in b are relative to WT-WAT by one-way analysis of variance (Dunnet's multiple comparison test) and significance is indicated as * P <0.05 and *** P <0.001. Full size image EpoR −/− -mice that die in utero due to disruption of definitive erythropoiesis [8] are rescued by the erythroid-expressing TgEpoR E transgene ( Tg -mice) that restores erythropoiesis. Although Tg -mice show no gross developmental or morphological defect, we show here that they exhibit abnormally increased weight gain from the first week after birth. By 10 months, the body weight of Tg -mice exceeded that of WT-mice by 60% in females and 30% in males. The greater accelerated weight gain in female Tg -mice may be related to estrogen-dependent Epo production that has been implicated in oestrus cycle-dependent uterine angiogenesis [23] . The excessive body weight in Tg -mice was due to increased white fat mass since neither brown fat nor lean mass were altered, suggesting an obese phenotype. Accompanying the disproportionate white fat accumulation was deterioration of insulin sensitivity, evident by 4 months in female mice and 6 months in male mice. These results link Epo activity in non-haematopoietic tissues to white fat mass accumulation and propose an effect of endogenous Epo in maintaining normal fat mass. Haematocrit and weight gain in EpoR +/− -mice with or without the TgEpoR E transgene were indistinguishable from WT-mice providing evidence that the increase of weight gain in Tg -mice is a consequence of loss of EpoR expression in non-haematopoietic tissue rather than transgene-related. Red cell production seemed normal in Tg -mice and Epo treatment in both WT- and Tg -mice increased haematocrit. However, only WT-mice exhibited the decreased fat mass compared with saline-treated control mice. In ob/ob -mice with Epo treatment, phlebotomy prevented the increase of haematocrit but did not affect the Epo-induced decrease of body weight gain in these mice. These data demonstrate that the regulatory effect of Epo on fat mass accumulation is independent of erythropoiesis. Decreased total activity and rate of oxygen consumption in Tg -mice was detected at 2 months, before the massive increase in fat mass. In contrast, Epo treatment in HFD-fed WT-mice reduced fat mass accumulation, increased total activity and reduced food intake. These changes as consequences of alteration in Epo signalling indicate a breakdown of energy homeostasis leading to disruption of stability in body fat storage. Rodents and humans exposed to high altitude exhibit decreased food intake, loss of body fat with accompanying decreased plasma glucose and insulin [24] , [25] . It is tempting to speculate that hypoxia inducible Epo may contribute to hypophagia and loss of body fat associated with high altitude. The hypothalamus is an organ responsible for regulating energy metabolism. Two populations of neurons in the arcuate nucleus of hypothalamus act in an opposing manner to control of food intake, energy expenditure and glucose metabolism. POMC-expressing neurons sense the change in peripheral regulatory hormones, leptin and insulin, and respond by secreting α-melanocyte-stimulating hormone that stimulates melanocortin 3 and 4 receptors in target neurons to decrease food intake and increase energy expenditure [26] , [27] . Activation of NPY/ARGP neurons expressing orexigenic neuron peptides NPY and AGRP stimulates orexigens MCH and orexins expression in lateral hypothalamus target neurons to increase food intake and decrease energy expenditure [26] , [27] , [28] . Surprisingly, we observed high level of EpoR expression in murine hypothalamus localized to POMC neurons, and Epo regulated POMC expression but not anabolic hypothalamic neuropeptide expression. Furthermore, decreased POMC expression due to lack of Epo signalling in Tg -mice hypothalamus is consistent with decreased energy expenditure, increased metabolic efficiency and development of obesity. Increased POMC expression induced by Epo treatment provides an explanation for the decreased food intake, increased energy expenditure and decreased metabolic efficiency. These results show that Epo regulates energy homeostasis at least through its target, POMC neurons, in the hypothalamus. However, Tg -mice with 50% POMC expression are not hyperphagic and the development of obesity is more gradual than that in Pomc −/− mice reflecting a POMC-dose-dependent effect [29] . Recent observations of weight gain regulation and HFD-induced leptin resistance by PPARγ in the CNS [30] , [31] suggest additional possible mechanisms for Epo action, given the effect of Epo on PPARγ in WAT and in differentiating preadipocytes. However, PPARγ activity in the rat hypothalamus localized to the paraventricular nucleus [31] and not in the arcuate nucleus where we localize EpoR expression in POMC neurons. The high level of EpoR expression in WT-WAT and the obese phenotype in Tg-mice that lack EpoR expression in WAT led us to explore Epo activities during preadipocyte proliferation and differentiation. Epo binding to the EpoR homodimer in erythroid progenitor cells activates Janus kinase 2 and downstream ERK and p38MAPK signalling pathways [5] , [6] , [7] , [32] . Similarly, Epo activates ERK and p38MAPK in differentiating preadipocytes, consistent with reports of ERK activity increasing PPARγ phosphorylation and decreasing PPARγ activity [19] , [33] . Adipocyte number is largely established during childhood and adolescence [34] . A recent study also suggests that early adipocyte progenitor cell number has a critical role in fat mass determination [35] . Epo treatment during preadipocyte differentiation decreased the terminal expansion of cell number following MDI induction and reduced preadipocyte differentiation. This is consistent with expansion of growth-arrested 3T3-L1 cells during differentiation induction as a critical step for subsequent adipogenic gene expression and adipocyte phenotype decision [36] . The effect of Epo in reducing the cell number of differentiating preadipocytes suggests that loss of Epo activity in WAT may result in an increase of the total adipocyte number. Indeed, Tg -WAT exhibits marked increase in fat cell number and decrease in fat cell size despite the disproportionate increased fat mass accumulation. Mice homozygous for a PPARγ-2 phosphorylation site mutation (S112A) show a WAT phenotype of greater number and smaller size of adipocytes compared with WT-WAT [37] , indicating that reduced or absent phosphorylation of PPARγ-2 can lead to increased fat cell number in vivo [36] . Similarly, endogenous Epo signalling in WAT may contribute to regulation of the adipocyte number. Multiple hormones including insulin, leptin and adiponectin regulate food intake and energy expenditure through the CNS [17] , [21] . Plasma insulin was significantly elevated in Tg -mice when their obese phenotype became noticeable, suggesting that insulin resistance may be a consequence of obesity in Tg -mice. Serum leptin and adiponectin levels appear proportional to fat content—elevated with increased fat mass in Tg -mice, and reduced with decreased fat mass in Epo-treated WT-mice. Both leptin and adiponectin mRNA level in WAT are comparable between WT- and Tg -mice. Epo treatment in WT-MEF cell cultures shows no effect in regulation of leptin and adiponectin gene expression both before and after differentiation. In addition, Epo treatment significantly reduced fat mass in leptin-deficient ob/ob -mice, indicating that leptin signalling may contribute but is not required for Epo regulation of body weight. Adiponectin is implicated in regulation of gluconeogenesis, fatty acid oxidation, food intake and energy expenditure by stimulating AMP-activated protein kinase and peroxisome proliferator-activated receptor-α [18] , [38] , and declines in obese patients and animal models that are insulin resistant, suggesting that decreased adiponectin level contributes to development of obesity and insulin resistance [39] . However, serum adiponectin levels in young Tg -mice with modest obesity before onset of insulin resistance were higher than those in control WT-mice. Hence, adiponectin is an unlikely causal factor of obesity and insulin resistance in Tg -mice. However, EpoR expression is elevated in WAT from obese WT-mice and ob/ob -mice and we observed an increase expression of proinflammatory adipokines in Tg - and ob/ob -WAT and reduced IL-10 in Tg -WAT. The improved insulin resistance with Epo treatment in ob/ob -mice and WT-mice on HFD may relate to the immune-modulatory effects associated with Epo [40] in non-haematopoietic tissue that is absent in Tg -mice. Reports of Epo-stimulated activation of an EpoR interaction with the GM-CSF/IL-3/IL-5 receptor common β-chain in haematopoietic and non-haematopoietic cells or tissues raised the possibility of an alternate Epo receptor [41] , [42] , [43] . The studies presented here do not directly address the nature of the non-haematopoietic Epo receptor. However, the relatively high level of EpoR expression that we observed in the hypothalamus and WAT is consistent with the hypothesis that EpoR expression level determines Epo response and formation of the “classical” EpoR in these non-haematopoietic tissues. While the essential role of Epo in erythropoiesis has been well established, the biological activity of Epo in non-haematopoietic tissues remains poorly understood. In the current study, we found significant EpoR expression in WAT and hypothalamus. Epo regulates POMC expression in hypothalamus and ablation of Epo signalling in hypothalamus disrupts energy homeostasis and leads to development of obesity and insulin resistance in Tg -mice. The effects of Epo in suppressing preadipocyte differentiation in vitro are associated with increased PPARγ phosphorylation and reduced preadipocyte expansion during differentiation. The lack of Epo signalling in WAT results in an increase in adipocyte number, which may lead to predisposition to this central defect-driven obesity. Together, these data indicate a role of Epo in maintaining normal fat mass in mice and suggest that further investigations are warranted to fully understand the central regulation of Epo in energy homeostasis. Animals Tg -mice containing the TgEpoR E transgene (GATA-1 locus haematopoietic regulatory domain driving mouse EpoR cDNA [12] ) were established on the EpoR −/− (C57BL/6) background (Jackson Laboratories) to obtain EpoR −/− TgEpoR E -mice. Heterozygous EpoR +/− -mice and EpoR +/− TgEpoR E -mice with the transgene were generated. Genotypes were identified by PCR (Neo gene (339 bp), WT EpoR (387bp) and transgene (303 bp)) ( Supplementary Table S1 ). Mice including WT-mice (C57BL/6), ob/ob -mice (Jackson Laboratories) and lean littermate control-mice were maintained on a 12-h light/dark cycles and fed regular chow NIH-07 diet (Zeigler Brothers) or HFD D12451 (Research Diets Inc.) as indicated. Animal procedures following National Institutes of Health guidelines were approved by NIDDK Animal Care and Use Committee. The mouse strains and the number, gender and age are listed in Supplementary Table S2 . Body weight and composition Body weight was measured using the same balance by the same person. Body composition was measured using the EchoMRI 3-in-1 (Echo Medical Systems). CT for fat determination X-ray CT (MicroCat II, Imtek) was used for imaging rodents at 50–100 μ resolutions under anaesthesia. Three-dimensional reconstructions of microCT images utilized the Hamming algorithm for soft tissue and semi-automatic algorithms to identify fat by anatomic sites (visceral, subcutaneous and nuchal-scapular brown fat) with the established Hounsfield Units. Amira 4.1 software for three-dimensional image analysis (Mercury ComputerSystems) was used to determine the total volume for each fat type. Epo treatment with haematocrit measurement For Epo treatment (3000 U kg −1 ; Epoetin alpha, Amgen Manufacturing), mice received intraperitoneal injection three times per week. Haematocrit was measured manually before and every week after Epo application. Serum parameter analyses Triglycerides were determined using Infinity Triglycerides reagents (Thermo DMA). Insulin, leptin and adiponectin concentrations were determined by radioimmunoassay (Linco Research). Glucose tolerance test and insulin tolerance test Mice fasted overnight were injected intraperitoneally with glucose (2.0 g kg −1 body weight) or insulin (humulin R, 0.75 mU kg −1 ). Blood glucose levels were measured before (0 min) and up to 120 min after the injection (3 μl from tail vein; Elite Glucometer (Bayer)). For determination of insulin secretion in response to glucose stimulation, 30 μl of blood was collected before (0 min) and up to 120 min after glucose injection; serum was prepared and frozen on dry ice immediately for later assessment. Open-field assay Spontaneous locomotor and explorative activities were measured using an open-field system (AccuScan Instruments, 8″×8″ configuration). Mice are tested between 6:00 and 11:00 for 3 consecutive days. Data were recorded for 60 min after 10 min acclimation to new environment and are expressed as averages from 3 days of testing. Indirect calorimetry and food intake Indirect calorimetry including oxygen consumption and activity measurements were assessed [44] . Oxygen consumption and CO 2 production were measured at 24 C° every 20 min for 47 h using an eight-chamber Oxymax System (Columbus Instruments; 2.5 l chambers with wire mesh floors and gauze as bedding, using 0.6 l min −1 flow rate, 90 s purge and 30 s measure; one mouse per chamber). The system was calibrated using a defined mixture of O 2 and CO 2 . Mice were allowed to adapt to individual housing for 3 weeks. During testing food and water were provided ad libitum . Motor activities were determined by infrared beam interruption (Opto-Varimex mini; Columbus). Resting metabolic rate was calculated with ambulation equal zero. The respiratory exchange ratio was calculated as the ratio between VCO 2 and VO 2 . Data were expressed as averages of 46 h excluding the first hour of the experiment. Oxygen consumption data were normalized to (body weight) 0.75 . Real-time reverse transcription (RT)–PCR Total RNA extracted from cells or tissues using TRIzol (Invitrogen) was treated with Turbo DNase (Ambion) and 2 μg was reverse transcribed (MultiScribe Reverse Transcriptase (ABI)) for quantitative PCR assays. Relative mRNA quantification of adipokine genes used Taqman gene expression assays (Invitrogen, Supplementary Table S3 ). For absolute quantification of mouse EpoR mRNA in fat and hypothalamus, probe-based Taqman PCR and mouse EpoR and S16 cDNA plasmid were used (S16, internal control). For relative mRNA quantification of all other genes, SYBR green real-time RT–PCR was used with normalization to house keeping genes β-actin and 18S using the delta-delta CT method. Primers and probes used in Taqman PCR and SYBR green real-time RT–PCR are listed in Supplementary Table S4 . Preparation of primary neonatal cardiomyocytes Hearts from postnatal 1-day mice were finely minced. Tissue was digested with collagenase/pancreatin at 37 °C for 10 min, disrupted by gently pipetting (10×), and the supernatant was transferred into cold PBS with 50% fetal bovine serum (FBS). After three cycles of digestion, cells were plated in cardiomyocyte culture medium SmGM-2 medium (CC3181 and CC4149, Lonza), non-adherent cells (cardiomyocytes) were collected after 40 min and replated into collagen I coated dishes. Fractionation of cells from WAT Inguinal fat pads were collected, digested with 1 mg ml −1 collagenase (type II) (37 °C, 50 min) and the reaction was stopped with equal volume of 50% FBS in DMEM. After centrifugation (600 g , 10 min), floating mature adipocytes were separated from the pellet of stromal vascular cells. Cells were plated and analysed after 24 h. Measurement of fat cell size Cell-size distribution was measured in gonadal fat pad from Tg - and WT-mice using Beckman Coulter Multisizer III [45] . Tissue samples from multiple areas and critically the same locations in each fat pad were immediately fixed in osmium tetroxide (37 °C, 48 h), and adipose cell size was determined with a 400-μm aperture (20–240 μm cell size range). In all, 6,000 events were counted for each sample. Preparation of MEF cells Embryos at day 14 post coitum (brain and dark red organs removed) were finely minced and digested with trypsin-EDTA (Gibco 25300) (37 °C) at 1 ml per embryo with gentle shaking for 30 min (gentle disruption pipetting up and down 10× every 10 min), and the reaction stopped with equal volume of cold PBS with 50% FCS. The solution was filtered (Falcom 40 mm cell strainer) and cells were collected by centrifugation, washed twice with fresh MEF culture medium (DMEM-high glucose, 10% FBS, 1% pen/strep, Gibco), suspended in warm MEF culture medium and plated (one embryo per dish). Medium was changed at 1 h to remove the unattached cells. Remaining cells were cultured and then frozen for later use. Preadipocyte differentiation MEF cells and 3T3-L1 cells (American Type Culture Collection) were grown in 10% CO 2 , in DMEM, 10% FBS, 1% pen/strep (Gibco). For preadipocyte differentiation, cells at 100% confluency were stimulated in DMEM medium supplemented with 0.5 mM 3-isobutyl-1-methylxanthine, 5 μg ml −1 insulin and 1 μM dexamethasone (Sigma) in the absence or presence of Epo. After 3 days, maintenance medium (DMEM, 10% FBS, 1% pen/strep, 5 μg ml −1 insulin) was used and changed every day. Fresh Epo was added at medium changes. Oil red O staining After preadipocyte differentiation, cells were washed with PBS gently and fixed (10% formalin, 1 h, room temperature). Formalin was removed and fresh oil red O solution (0.3% in 60% isopropanol) was added to stain the cells (1 h, gentle swirling). Cells were rinsed with distilled water thoroughly. For quantification, stained dishes were dried, oil red O was resuspended in isopropanol (1 min) and solution OD was determined at 510 nm. Western blotting WAT and MEF cells were homogenized, incubated in lysis buffer (50 mM Tris–HCI buffer, pH 7.4, 1% NP40, 150 mM NaCl, 1 mM EDTA, 1% Triton X-100, 0.1% SDS, 1% sodium deoxycholate) with phosphotase and proteinase inhibitors (Roche) (30 min on ice), and cell debris was removed by centrifugation. Protein concentration was determined using Pierce BCA protein assay kit (Thermo Scientific). Sample proteins (30 μg for each) were electrophoretically separated, blotted using XCell SureLock Mini-Cell system (Invitrogen) ( Supplementary Information ) and visualized using protein-specific antibodies ( Supplementary Table S5 ) and the Amersham ECL Advance Western Blotting Detection System (GE Healthcare Bio-Sciences Corp). Quantitative analysis was performed by measuring integrated density with the NIH image J system and normalized with β-actin. Fluorescent immunohistochemistry After dewaxing and rehydration, antigen retrieval was performed by autoclaving using antigen-unmasking solution (Vector Laboratories). Rabbit anti-mouse POMC antibody (kindly provided by Dr Peng Loh; Cellular Neurobiology Section, NICHD/NIH) and FITC-conjugated goat anti-rabbit IgG (M30201, Invitrogen) as a secondary antibody were used for labelling POMC neurons. Concerns about commercial EpoR antibodies suggest caution regarding their use [46] , [47] . As we found variability among commercial lots of EpoR polyclonal antibody, we used the monoclonal antibody developed at Genetics Institute against the EpoR extracellular domain (mh2er/16.5.1) that previously provided consistent results for immunohistochemistry [48] , [49] and Alexa594-conjugated goat anti-mouse IgG (A11020, Invitrogen) in detecting mEpoR. Preparation of primary adult hypothalamic neurons Adult neurons were isolated from hypothalamus [50] and cultured for 24 h, then treated with Epo (5 U ml −1 ) or saline for 24 h. Total RNA were extracted and analysed for POMC, NPY, AGRP, prepro-orexin and pro-MCH gene expression. Statistical analysis The data are expressed as mean±s.e.m. Comparisons between two groups were made using two-tailed non-paired Student's t -test. Statistical differences between three or more groups were evaluated by one-way analysis of variance with Dunnet's multiple comparison post hoc tests at α =0.05. A P value of <0.05 was regarded to be statistically signicant. How to cite this article: Teng, R. et al . Disrupted erythropoietin signalling promotes obesity and alters hypothalamus proopiomelanocortin production. Nat. Commun. 2:520 doi: 10.1038/ncomms1526 (2011).